Autoprocessing of neutrophil elastase near its active site reduces the efficiency of natural and synthetic elastase inhibitors An imbalance between neutrophil-derived proteases and extracellular inhibitors is widely regarded as an important pathogenic mechanism for lung injury. Despite intense efforts over the last three decades, attempts to develop small-molecule inhibitors for neutrophil elastase have failed in the clinic. Here we discover an intrinsic self-cleaving property of mouse neutrophil elastase that interferes with the action of elastase inhibitors. We show that conversion of the single-chain (sc) into a two-chain (tc) neutrophil elastase by self-cleavage near its S1 pocket altered substrate activity and impaired both inhibition by endogenous α-1-antitrypsin and synthetic small molecules. Our data indicate that autoconversion of neutrophil elastase decreases the inhibitory efficacy of natural α-1-antitrypsin and small-molecule inhibitors, while retaining its pathological potential in an experimental mouse model. The so-far overlooked occurrence and properties of a naturally occurring tc-form of neutrophil elastase necessitates the redesign of small-molecule inhibitors that target the sc-form as well as the tc-form of neutrophil elastase. Neutrophil elastase is abundantly expressed by neutrophil precursors in bone marrow and stored in primary (azurophil) granules in its mature active form. During inflammation, NE is released into the extracellular space, where its activity is tightly contained by alpha-1-antitrypsin (AAT), an abundant neutrophil elastase inhibitor of blood plasma. Intratracheal instillation of human neutrophil elastase and porcine pancreas elastase into an animal model lead to emphysema and was the first indication that an imbalance between neutrophil elastase and AAT is an important pathogenic mechanism for lung injury [1] , [2] . Both environmental factors like cigarette smoke or air pollution and genetic factors can lead to a disruption of the protease–antiprotease balance [3] , [4] , [5] . While other locally acting elastase inhibitors, for example, secretory leukocyte protease inhibitor and elafin [6] , [7] , also provide some anti-elastase protection in humans, only decreased levels of plasma AAT are known to be associated with chronic lung disease. Inherited deficiency including the complete absence of AAT, in particular, is associated with emphysema and chronic obstructive pulmonary disease development indicating that intermittently unopposed neutrophil elastase activity can damage lung tissues [8] . Although augmentation therapy has been accepted as a treatment of AAT deficiency, less cost-intensive alternatives, in particular small-molecule inhibitors for neutrophil elastase, have failed in the clinic despite many efforts over the last three decades. During our characterization of mouse neutrophil elastase, we discovered a spontaneous conversion process of the single-chain (sc) form of neutrophil elastase into a specific two-chain (tc) form by self-cleavage near its S1 pocket. The tc neutrophil elastase showed altered substrate activity and inhibition by AAT as well as by a small-molecule inhibitor. While autoprocessing of neutrophil elastase decreased the inhibitory ability of AAT and synthetic small-molecule inhibitors, the pathological potential of tc neutrophil elastase was retained. The occurrence of the so-far unnoticed tc neutrophil elastase with its altered properties adversely affects the protease–antiprotease balance in the lung during neutrophil elastase release in response to external challenges and should be considered for the development of more efficient anti-elastase therapies. Identification of two internal cleavage sites At the high concentrations (estimates are up to 5 mM) immediately reached after granule secretion [9] , neutrophil elastase is able to nick itself, resulting in an altered activity of neutrophil elastase ( Fig. 1a ). This self-nicking activity was routinely observed in vitro already at much lower concentrations than 5 mM when the propeptide was removed by enterokinase. Conversion into the mature form was achieved as demonstrated by SDS–polyacrylamide gel electrophoresis (SDS–PAGE). Besides the mature sc-form of mouse neutrophil elastase, two bands (band 3 and 4) were generated in increasing amounts over time. Using Edman sequencing, we identified these bands as amino-terminal fragments of mouse neutrophil elastase starting with the mature N terminus, namely Ile16-Val17 ( Fig. 1b , chymotrypsinogen numbering according to Bode et al . [10] ). The predominant carboxyl-terminal fragment (outside the gel sections shown in Fig. 1 ) started at position 189 with Gly189, the minor fragment with Cys182 ( Fig. 1b ). Nicking of mouse neutrophil elastase also continued after adding an enterokinase specific inhibitor (DDDK-chloromethylketone) pointing to a self-cleavage of mature mouse neutrophil elastase. These bands did not appear, when we processed the catalytically inactive Ser195Ala variant of mouse neutrophil elastase under the same conditions ( Fig. 1c ). Cleavage after Ala188 preceded the cleavage at the minor nick site after Val181. Both nick sites are located on the surface and are consistent with the cleavage specificity of both human neutrophil elastase and mouse neutrophil elastase. The carboxyl-terminal fragments carrying the active site Ser195 cannot be released from the native molecule as the native structure of neutrophil elastase is stabilized by a conserved disulfide bond between Cys136 and Cys201 ( Fig. 1b ). 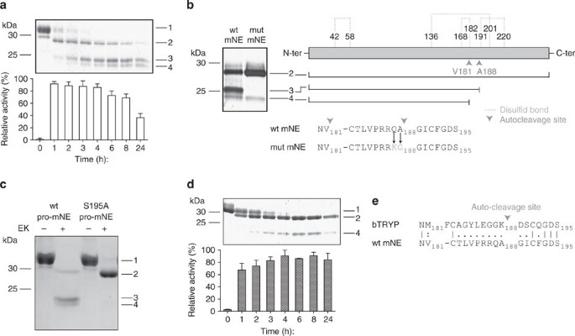Figure 1: Self-cleavage of mouse neutrophil elastase after activation. (a) At time zero, enterokinase (25–50 μg ml−1) was added to mouse neutrophil elastase (1–2 mg ml−1) and processing of the mouse neutrophil elastase zymogen was analysed over 24 h by SDS–PAGE and Coomassie blue staining. Activity at the same points in time were recorded using Abz-GAVVASELR-Y(NO2)-D as a fluorogenic substrate. Data shown are the mean±s.e.m. of all experiments (n=5) and was normalized to the time point (100%) showing the highest activity. Self-cleavage of mouse neutrophil elastase started immediately and continued even in the presence of an enterokinase specific inhibitor (not shown). Activity declined in particular with the appearance of band 3 and 4 of the tc neutrophil elastase. (b) Autoprocessed mouse neutrophil elastase (mNE;b, lane 1) was blotted onto Immobilon PVDF membrane after SDS–PAGE (18% polyacrylamide Tris tricine gel) and the two low molecular weight bands (outside of the gel section depicted) were analysed by Edman sequencing. The N terminus of these fragments started with sequences (grey arrow heads) shown in the alignment of wild-type murine neutrophil elastase (wt mNE, middle row) and the mutated murine NE (mut mNE). Replacement of Gln187–Ala188 by Lys187–Gly188 as found in azurocidin prevents the formation of band 3, the major tc-form (right lane, mut mNE). (c) Recombinant wt mNE and inactive mutant S195A mNE (0.47 mg ml−1) were incubated with enterokinase EK (15 μg ml−1) at 37 °C for 24 h. Tc-mNE was only found with active wt mNE. (d) The experimentawas repeated with mut mNE. Data shown are the mean±s.e.m. of all experiments (n=5) and was normalized to the time point (100%) showing the highest activity. Mut mNE shows some minor autoprocessing activity for the second internal site, but a highly stable activity for more than 24 h after enterokinase-mediated conversion of its zymogen. (e) Bovine cationic trypsin (bTRYP, upper row) was aligned with mNE. The self-cleavage position of the so-called pseudotrypsin with chymotrypsin-like activity is indicated by the grey arrow head pointing downward. C-ter, C-terminal; N-ter, N-terminal. Figure 1: Self-cleavage of mouse neutrophil elastase after activation. ( a ) At time zero, enterokinase (25–50 μg ml −1 ) was added to mouse neutrophil elastase (1–2 mg ml −1 ) and processing of the mouse neutrophil elastase zymogen was analysed over 24 h by SDS–PAGE and Coomassie blue staining. Activity at the same points in time were recorded using Abz-GAVVASELR-Y(NO2)-D as a fluorogenic substrate. Data shown are the mean±s.e.m. of all experiments ( n =5) and was normalized to the time point (100%) showing the highest activity. Self-cleavage of mouse neutrophil elastase started immediately and continued even in the presence of an enterokinase specific inhibitor (not shown). Activity declined in particular with the appearance of band 3 and 4 of the tc neutrophil elastase. ( b ) Autoprocessed mouse neutrophil elastase (mNE; b , lane 1) was blotted onto Immobilon PVDF membrane after SDS–PAGE (18% polyacrylamide Tris tricine gel) and the two low molecular weight bands (outside of the gel section depicted) were analysed by Edman sequencing. The N terminus of these fragments started with sequences (grey arrow heads) shown in the alignment of wild-type murine neutrophil elastase (wt mNE, middle row) and the mutated murine NE (mut mNE). Replacement of Gln187–Ala188 by Lys187–Gly188 as found in azurocidin prevents the formation of band 3, the major tc-form (right lane, mut mNE). ( c ) Recombinant wt mNE and inactive mutant S195A mNE (0.47 mg ml −1 ) were incubated with enterokinase EK (15 μg ml −1 ) at 37 °C for 24 h. Tc-mNE was only found with active wt mNE. ( d ) The experiment a was repeated with mut mNE. Data shown are the mean±s.e.m. of all experiments ( n =5) and was normalized to the time point (100%) showing the highest activity. Mut mNE shows some minor autoprocessing activity for the second internal site, but a highly stable activity for more than 24 h after enterokinase-mediated conversion of its zymogen. ( e ) Bovine cationic trypsin (bTRYP, upper row) was aligned with mNE. The self-cleavage position of the so-called pseudotrypsin with chymotrypsin-like activity is indicated by the grey arrow head pointing downward. C-ter, C-terminal; N-ter, N-terminal. Full size image Inactivation by a second internal cleavage Using the same extended peptide sequence Abz-GAVVASELR-Y(NO2)-D as a substrate and normalizing all measurements to the highest activity in each experiment ( n =3), we still detected high activity for the tc-form of neutrophil elastase ( Fig. 1a ) although somewhat less than with sc neutrophil elastase ( Fig. 1d ). Internal cleavage of neutrophil elastase, therefore, did not inactivate this enzyme by contrast to a degradation-sensitive variant (Gly186Arg, chymotrypsinogen number) of anionic trypsin, which inactivates itself by cleavage at a slightly different topological position [11] . To confirm the catalytic activity of the tc-form, we incubated it with a biotinylated tetrapeptide chloromethylketone that forms an irreversible covalent bond with the histidine residue of the catalytic triad in active serine proteases [12] . As shown in Fig. 2 , both variants of the tc-form (corresponding to band 3 and band 4 of Fig. 1a ) were labelled with this activity-dependent suicide inhibitor. On closer inspection, the shorter amino-terminal fragment, however, appeared to have reacted only partially in comparison with the amounts of the two other forms present in this preparation ( Figs 2a and b , right lane). The non-reactive fraction most likely represents elastase molecules with two internal cleavages ( Figs 2c, b and 4 ). This finding is consistent with a moderate loss of elastase activity after prolonged incubation times when both the sc-form and the tc-variant 1 had declined in quantity ( Fig. 1a ). 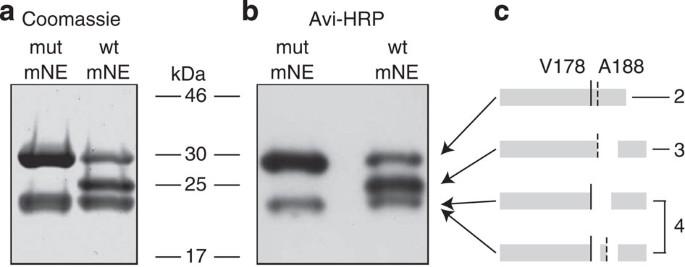Figure 2: Double internal cleavages appear to inactivate neutrophil elastase. Neutrophil elastase was incubated with biotinylated AAPV-chloromethylketone (neutrophil elastase inhibitor) at 37 °C for 30 min. (a) Eight μg of wild-type or mutated mouse neutrophil elastase (wt mNE or mut mNE) was separated by SDS–PAGE and stained with Coomassie blue. There were equal amounts of band 3 and 4. (b) One μg of each mouse neutrophil elastase form was separated by SDS–PAGE and analysed by western blotting using avidin-HRP. The signal for band 3 was much stronger compared with band 4. (c) Scheme showing the molecular structure of the three neutrophil elastase bands. The lowest band (4) contains single-nicked mouse neutrophil elastase as well as double-nicked mouse neutrophil elastase. The double-nicked mouse neutrophil elastase does not appear to react with the chloromethylketone as judged from the reduced western blot signal (b) in comparison with the total amount of the tc neutrophil elastase (a). The experiment was repeated thrice. Figure 2: Double internal cleavages appear to inactivate neutrophil elastase. Neutrophil elastase was incubated with biotinylated AAPV-chloromethylketone (neutrophil elastase inhibitor) at 37 °C for 30 min. ( a ) Eight μg of wild-type or mutated mouse neutrophil elastase (wt mNE or mut mNE) was separated by SDS–PAGE and stained with Coomassie blue. There were equal amounts of band 3 and 4. ( b ) One μg of each mouse neutrophil elastase form was separated by SDS–PAGE and analysed by western blotting using avidin-HRP. The signal for band 3 was much stronger compared with band 4. ( c ) Scheme showing the molecular structure of the three neutrophil elastase bands. The lowest band (4) contains single-nicked mouse neutrophil elastase as well as double-nicked mouse neutrophil elastase. The double-nicked mouse neutrophil elastase does not appear to react with the chloromethylketone as judged from the reduced western blot signal ( b ) in comparison with the total amount of the tc neutrophil elastase ( a ). The experiment was repeated thrice. Full size image Conserved self-cleavages in neutrophil elastase and trypsin Self-cleavage of the same loop in another serine protease, bovine cationic trypsin, has been described in the 1960s resulting in a functionally active new trypsin species with altered chymotrypsin-like activity, called pseudotrypsin [13] . The critical self-cleavage at Lys176/Asp177 (Lys188/Asp189, numbered according to chymotrypsinogen) [13] occurred at the same topological position, as in mouse neutrophil elastase between Ala188/Gly189 ( Fig. 1e ). Mass spectrometry-grade trypsins from commercial sources are chemically methylated at Lys188 and thereby retain their strict Arg/Lys specificity. Although the surface loop 185 through 188 does not directly contact the substrate, it plays a significant role in determining substrate specificity [14] . To prove this particular position 188 as the critical target for limited proteolysis in mouse neutrophil elastase, we replaced the Gln187–Ala188 dipeptide with Lys187–Gly188 as found in human azurocidin [15] , and successfully eliminated the self-processing of natural mouse neutrophil elastase ( Fig. 1b ). By repeating the experiment shown in Fig. 1a , we were able to verify that this mutated mouse neutrophil elastase was stable and kept its activity even after 24 h ( Fig. 1d ). Tc neutrophil elastase found in human and murine neutrophils Identical residues at position 188 and 189, namely Ala–Gly, occur in many mammalian neutrophil elastase homologues and are expected to trigger a natural autodigestive modification of neutrophil elastase in general. Accordingly, the tc neutrophil elastase was found in both murine and human polymorphonuclear neutrophil (PMN) lysates ( Fig. 3 ). Freshly isolated murine and human PMNs were quickly lysed in reducing SDS sample buffer and boiled to avoid any autodegradation of mouse neutrophil elastase during lysate preparation. The expected mouse neutrophil elastase band at 27 kDa and the two bands around 19 kDa are found in wild type, but not in PR3/NE double-deficient PMN lysate [16] confirming the specificity of the antibodies. Haptoglobin served as a loading control [17] . In contrast to mouse PMNs, human PMNs were lysed in the presence of a biotinylated AAPV-chloromethylketone, an irreversible activity-based inhibitor of both proteinase 3 and neutrophil elastase. The covalently biotinylated neutrophil elastase was then immunoprecipitated with a monoclonal antibody specific for human neutrophil elastase and visualized after SDS–PAGE and western blotting using streptavidin-peroxidase. Our analyses conclusively demonstrate that self-processing of neutrophil elastase occurs rapidly even with careful preparation of unstimulated neutrophils from murine bone marrow cells ( Fig. 3a ) and peripheral blood leukocytes ( Fig. 3b ). Human neutrophil elastase preparations made from sputum material also showed a similar pattern of fragmentation when biotinylated AAPV-chloromethylketone was added indicating that proteolytically modified neutrophil elastase is present in biological fluids and retains its activity under these conditions ( Fig. 3b ). 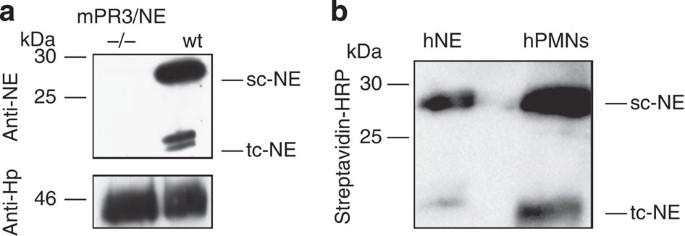Figure 3: The tc- and sc-form of neutrophil elastase in human and murine neutrophils. (a) Mouse neutrophils were purified from bone marrow cells. Total cell lysates were analysed by SDS–PAGE and western blotting using an anti-neutrophil elastase polyclonal antibody. To demonstrate the specificity of the antibody for neutrophil elastase, lysates from PR3/NE double-knockout mice were processed in the same way and absence of similar immunoreactive fragments was verified (left lane). (b) Human PMNs were isolated from peripheral blood leukocytes and incubated with a biotinylated tetrapeptide (AAPV) chloromethyl ketone inhibitor during lysis. After immunoprecipitation with an anti-human neutrophil elastase monoclonal antibody and SDS–PAGE followed by western blotting, active site-labelled human neutrophil elastase was visualized using horseradish peroxidase-conjugated streptavidin. Two bands co-migrating with the respective bands of a human neutrophil elastase preparation from sputum were active site labelled by the chloromethyl ketone indicating the occurrence of an active tc neutrophil elastase (tc-NE) in biological samples. Both experiments were repeated thrice. Figure 3: The tc- and sc-form of neutrophil elastase in human and murine neutrophils. ( a ) Mouse neutrophils were purified from bone marrow cells. Total cell lysates were analysed by SDS–PAGE and western blotting using an anti-neutrophil elastase polyclonal antibody. To demonstrate the specificity of the antibody for neutrophil elastase, lysates from PR3/NE double-knockout mice were processed in the same way and absence of similar immunoreactive fragments was verified (left lane). ( b ) Human PMNs were isolated from peripheral blood leukocytes and incubated with a biotinylated tetrapeptide (AAPV) chloromethyl ketone inhibitor during lysis. After immunoprecipitation with an anti-human neutrophil elastase monoclonal antibody and SDS–PAGE followed by western blotting, active site-labelled human neutrophil elastase was visualized using horseradish peroxidase-conjugated streptavidin. Two bands co-migrating with the respective bands of a human neutrophil elastase preparation from sputum were active site labelled by the chloromethyl ketone indicating the occurrence of an active tc neutrophil elastase (tc-NE) in biological samples. Both experiments were repeated thrice. Full size image Altered substrate activity of the tc neutrophil elastase To search for a potential change of cleavage activity, preparations of the tc mouse neutrophil elastase and sc mouse neutrophil elastase were incubated with fluorescence resonance energy transfer peptides derived from the reactive centre loop sequences of AAT [18] , [19] and serpinB1 (MNEI) [20] , the most relevant mechanism-based inhibitors of neutrophil elastase in the extracellular and cytosolic compartment, respectively ( Table 1 ). The primary effect of intramolecular self-cleavage was a 12.5-fold decrease in the catalytical constant ( k cat ), while the Michaelis constant ( K m ) was marginally changed for the hydrolysis of the AAT peptide sequence. A different consequence has been found with the MNEI-derived peptide, its K m was fivefold lower, indicating that the serpinB1-derived peptide was binding fivefold more tightly, but its k cat value was 29-fold lower. The k cat values characterize the rate of product formation encompassing an acylation and deacylation step which both could be impaired. Studying the interaction between neutrophil elastase and a pseudosubstrate, AAT, with the formation of a covalent acyl complex, should give us a clue as to whether acylation was affected by the internal cleavage modification. Table 1 Autocleavage of mouse neutrophil elastase changed substrate specificity. Full size table Impaired inhibition of tc neutrophil elastase by AAT We, therefore, analysed the kinetics of complex formation between the sc- and tc-form of mouse neutrophil elastase and AAT. As shown in Table 2 , the association rate constant of AAT with the tc-form was 10-fold slower than that of sc neutrophil elastase. This difference in AAT reactivity was further confirmed by Coomassie Brilliant Blue staining of the protein bands after SDS–PAGE ( Fig. 4 ). Complexes between the sc- and the tc-form can be easily distinguished by their size difference, as a covalent complex is formed between the active site serine of neutrophil elastase Ser195 and the methionine carboxyl group of the reactive centre loop of AAT Met358. Reactivity with the tc-form is visualized by the appearance of a band slightly larger than native AAT, while the complex between the sc neutrophil elastase and AAT is easily recognized as a 80-kDa band. The tc-related complex is formed significantly slower than the 80-kDa complex in the presence of a partially nicked wild-type neutrophil elastase. Table 2 Impaired inhibition of tc-NE. 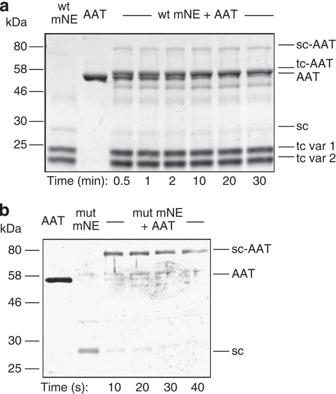Figure 4: Impaired inhibition of tc mouse neutrophil elastase by AAT. Wild-type or mutated mouse neutrophil elastase (wt mNE or mut mNE) was mixed with AAT at a ratio of 2:3 and incubated at 37 °C. A covalent bond is formed between the Ser195 of neutrophil elastase and the Met358 of AAT. To study the complex formation over time, aliquots were withdrawn at the indicated time points and analysed by SDS–PAGE and Coomassie staining. (a) The tc neutrophil elastase–AAT complex (tc-AAT) is smaller than the sc neutrophil elastase–AAT complex (sc-AAT) as only the small 7-kDa carboxyl-terminal fragment of tc mouse neutrophil elastase remains covalently bound to AAT in reducing conditions. While sc neutrophil elastase–AAT complexes form within seconds, tc neutrophil elastase–AAT complex formation takes several minutes. (b) Mutated mouse neutrophil elastase consists of almost exclusively sc neutrophil elastase. The reaction with AAT is finished after ten seconds. Both experiments were repeated thrice. Full size table Figure 4: Impaired inhibition of tc mouse neutrophil elastase by AAT. Wild-type or mutated mouse neutrophil elastase (wt mNE or mut mNE) was mixed with AAT at a ratio of 2:3 and incubated at 37 °C. A covalent bond is formed between the Ser195 of neutrophil elastase and the Met358 of AAT. To study the complex formation over time, aliquots were withdrawn at the indicated time points and analysed by SDS–PAGE and Coomassie staining. ( a ) The tc neutrophil elastase–AAT complex (tc-AAT) is smaller than the sc neutrophil elastase–AAT complex (sc-AAT) as only the small 7-kDa carboxyl-terminal fragment of tc mouse neutrophil elastase remains covalently bound to AAT in reducing conditions. While sc neutrophil elastase–AAT complexes form within seconds, tc neutrophil elastase–AAT complex formation takes several minutes. ( b ) Mutated mouse neutrophil elastase consists of almost exclusively sc neutrophil elastase. The reaction with AAT is finished after ten seconds. Both experiments were repeated thrice. Full size image Impaired inhibition of tc-elastase by a synthetic inhibitor Proteolytic modification at this position in neutrophil elastase should similarly impair the inhibitory efficiency of small synthetic chemicals. Because of their advantages for therapeutic applications, non-electrophilic reversible inhibitors have recently been optimized for high-affinity binding to human neutrophil elastase. One of these compounds, named AZ11777736, was kindly provided to us by AstraZeneca (Mölndal, Sweden). As expected, we not only noticed a 10-fold decline in the association rate constant between AAT and the tc mouse neutrophil elastase, but also a 14-fold increase in the dissociation constant of this small-molecule inhibitor and the tc mouse neutrophil elastase compared with sc neutrophil elastase ( Table 2 ). Pathogenicity of the tc-form of mouse neutrophil elastase The basic experiment leading to the protease–antiprotease concept was the intratracheal instillation or aerosol inhalation of purified proteases in animal models including papain, porcine pancreatic elastase, human PR3 or human neutrophil elastase [1] , [2] . All these proteases, however, have different cleavage specificities and affinities for endogenous mouse inhibitors [21] , [22] , [23] , [24] . To overcome these experimental limitations, we applied and evaluated for the first time mouse neutrophil elastase as an experimental inducer of lung emphysema and also considered the tc-form of neutrophil elastase as a potential pathogenic trigger in vivo . Our in vivo experiments with quantitative assessment of airspace enlargement ascertained the pathogenic role of the endogenous murine homologue and, moreover, revealed that the autoprocessed form of mouse neutrophil elastase induced similar emphysema-like changes in mouse lung tissues as the sc-form after 2 months ( Fig. 5 ). Both forms, sc and tc neutrophil elastase, induced an inflammatory infiltrate of cells within 24 h, in particular, of macrophages and of neutrophils, but not of lymphocytes, which was verified by lung tissue staining and analysis of bronchoalveolar lavage (BAL) fluids ( Fig. 6a,b ). Compared with buffer controls, these cellular findings are paralleled by an upregulation of the chemokines MCP1/CCL2 and KC/CXCL2 at the RNA (data not shown) and protein level ( Fig. 6c ) attracting monocytes and neutrophils, respectively. 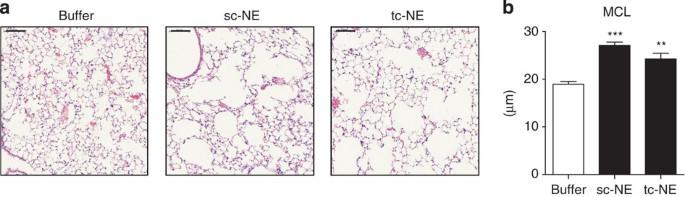Figure 5: Pathogenicity of the tc-form of mouse neutrophil elastase. (a) Representative micrographs of haematoxylin and eosin-stained lung tissue 2 months after a single oropharyngeal application of sc neutrophil elastase (sc-NE), tc neutrophil elastase (tc-NE) or buffer (300 mM NaCl, 20 mM Na2HPO4pH7.4; scale bars, 100 μm). (b) Unlike buffer-exposed mice, tc-NE and sc-NE treatment generated a marked airspace enlargement, confirmed by mean chord length (MCL) determination of buffer, sc-NE and tc-NE exposed mouse lungs. Data (mean±s.e.m.) are representative of two independent experiments withn=3 (buffer) andn=4 (sc- or tc-NE). One-way analysis of variance Bonferroni test was applied (**P<0.01, ***P<0.001). Figure 5: Pathogenicity of the tc-form of mouse neutrophil elastase. ( a ) Representative micrographs of haematoxylin and eosin-stained lung tissue 2 months after a single oropharyngeal application of sc neutrophil elastase (sc-NE), tc neutrophil elastase (tc-NE) or buffer (300 mM NaCl, 20 mM Na 2 HPO 4 pH7.4; scale bars, 100 μm). ( b ) Unlike buffer-exposed mice, tc-NE and sc-NE treatment generated a marked airspace enlargement, confirmed by mean chord length (MCL) determination of buffer, sc-NE and tc-NE exposed mouse lungs. Data (mean±s.e.m.) are representative of two independent experiments with n =3 (buffer) and n =4 (sc- or tc-NE). One-way analysis of variance Bonferroni test was applied (** P <0.01, *** P <0.001). 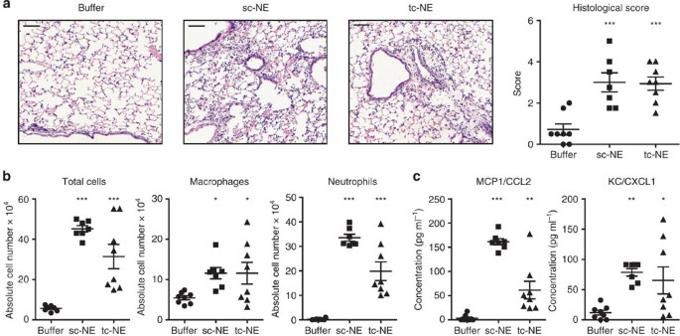Figure 6: Sc and tc mouse neutrophil elastase induce inflammation in lung. Mice were analysed 24 h after a single oropharyngeal application of sc neutrophil elastase (sc-NE), tc neutrophil elastase (tc-NE) or buffer (300 mM NaCl, 20 mM Na2HPO4pH7.4). (a) Representative micrographs of lung tissue were stained with haematoxylin and eosin (scale bars, 100 μm). The severity of inflammation was calculated using a five-point lung inflammation scoring system (0, no inflammation and 5, >30 inflammatory cells per field). Inflammation was more severe in mice treated with sc- or tc-mNE than buffer alone. (b) The amount of inflammatory cells in BAL was significantly increased in the BAL of sc- and tc-mNE-treated mice. Analysing May–Grünwald–Giemsa-stained cytospin slides revealed neutrophils as the main population followed by macrophages. (c) The protein level of two important chemokines MCP1/CCL2 and KC/CXCL1 were determined using ELISA. The sc- and tc-mNE-treated mice showed a significantly higher level of MCP1/CCL2 and KC/CXCL1 compared with buffer-treated mice. Data (mean±s.e.m.) are representative of two independent experiments with totaln=7 (sc-NE) andn=8 mice in the tc-NE and buffer control groups. One-way analysis of variance Bonferroni test was applied (*P<0.05, **P<0.01, ***P<0.001). Full size image Figure 6: Sc and tc mouse neutrophil elastase induce inflammation in lung. Mice were analysed 24 h after a single oropharyngeal application of sc neutrophil elastase (sc-NE), tc neutrophil elastase (tc-NE) or buffer (300 mM NaCl, 20 mM Na 2 HPO 4 pH7.4). ( a ) Representative micrographs of lung tissue were stained with haematoxylin and eosin (scale bars, 100 μm). The severity of inflammation was calculated using a five-point lung inflammation scoring system (0, no inflammation and 5, >30 inflammatory cells per field). Inflammation was more severe in mice treated with sc- or tc-mNE than buffer alone. ( b ) The amount of inflammatory cells in BAL was significantly increased in the BAL of sc- and tc-mNE-treated mice. Analysing May–Grünwald–Giemsa-stained cytospin slides revealed neutrophils as the main population followed by macrophages. ( c ) The protein level of two important chemokines MCP1/CCL2 and KC/CXCL1 were determined using ELISA. The sc- and tc-mNE-treated mice showed a significantly higher level of MCP1/CCL2 and KC/CXCL1 compared with buffer-treated mice. Data (mean±s.e.m.) are representative of two independent experiments with total n =7 (sc-NE) and n =8 mice in the tc-NE and buffer control groups. One-way analysis of variance Bonferroni test was applied (* P <0.05, ** P <0.01, *** P <0.001). Full size image In this study, a self-cleavage site at Ala188/Gly189 was identified in both recombinant as well as in native neutrophil elastase from PMNs. We studied autoprocessing of neutrophil elastase only in two mammalian species human neutrophil elastase and mouse neutrophil elastase, but as this combination of Ala–Gly at position 188 and 189 occurs in many mammalian species, autoprocessing of neutrophil elastase appears to be a general mechanism to regulate neutrophil elastase activity and specificity. Self-cleavage after residue Ala188 in neutrophil elastase occurs within a flexible loop of the activation domain of which Val190 and Phe192 affect the S1 subsite in neutrophil elastase [25] and influence interactions with substrates. As there was a 10-times decline in the association rate constant of neutrophil elastase with AAT after self-cleavage, we proved that cleavage of this loop affected the interaction of peptides with the substrate-binding region of neutrophil elastase and the association rate of AAT with the tc neutrophil elastase. A more direct indication for our suggestion that the S1 pocket was affected by autoprocessing is the 14-fold increase in the dissociation constant of a small-molecule inhibitor kindly provided by AstraZeneca. The key interaction of this non-covalently bound chemical (compound 10) [26] involves the deep insertion of the N -aryl group into the S1-binding pocket and additional hydrogen bonds between the pyridone and benzylamide moieties and neutrophil elastase (Peter Sjö, personal communication). These structural determinants of inhibitor binding are consistent with our observations of its reduced inhibitory activity on the tc-form of neutrophil elastase. Elevated local flexibility of the S1-binding groove evidently impairs the drug-target interplay and local dynamics of inhibitor recognition. Oropharyngeal application of sc and tc neutrophil elastase to mice showed that the pathogenic potential of NE was not lost after autoprocessing, and tc neutrophil elastase was still able to induce emphysema-like changes in mice. Direct comparisons of the effects of the sc-mutant and the tc-form for wild-type mouse neutrophil elastase, however, should be made with caution because of the lower stability of the tc-form during in vitro production and processing, The lower number of infiltrating cells and neutrophils ( Fig. 5b ) could be interpreted as a trend towards a slightly reduced pathogenicity of the tc-form, but the variability of the effects observed with it were relatively large compared with those of the sc-mutant. By contrast, macrophage levels in the BAL fluids did not differ between the sc- and the tc-elastase groups despite lower monocyte-recruiting CCL2 levels ( Fig. 5c ). Other monocyte-recruiting factors, for example, fragments of elastin [27] and of other matrix components, directly produced by the instilled elastase preparations, may be more relevant for tc neutrophil elastase-induced monocyte recruitment than CCL2 induction in this experimental model. As neutrophils are recruited at high densities to sites of invading bacteria or external noxious agents like cigarette smoke and nanoparticles, release of the proteolytically modified elastase from activated neutrophils, dying neutrophils and neutrophils engaged in frustrated phagocytosis should primarily contribute to the damage of lung tissues that are particularly exposed to environmental triggers, as seen in patients with AAT deficiencies. Up to now, small-molecule inhibitors were developed and optimized to target the sc-from of neutrophil elastase, as the existence of a post-translationally modified neutrophil elastase escaped attention or was simply ignored. Recognition of the tc neutrophil elastase as an additional pathogenic factor in neutrophil-mediated tissue damage necessitates the design of new inhibitors to target both NE forms with equal efficacy in the future. Expression and purification of proteins Mouse neutrophil elastase was amplified by the PCR from a complementary DNA clone. An artificial propeptide terminating in the sequence DDDK, an enterokinase cleavage site (DDDK), was fused to the N terminus of the mature elastase reading frame using the following oligoduplex DJ3385 5′Pho-CAG GTT CCA CTG GTA GCC GCA TGC ACC GCA ACG GCA GCC AC-3′ and DJ3386 5′-Pho-GTG GCT GCC GTT GCG GTG CAT GCG GCT ACC AGT GGA ACC TGG TAC-3′. To enable secretion, the Igκ-chain secretion signal was added with an oligoduplex, DJ2972 5′-Pho-CTA GCC ACC ATG GAG ACA GAC ACA CTC CTG CTA TGG GTA CTG CTG CTC TGG GTAC CAG GTT CCA C-3′ and DJ2973 5′-Pho-GT GGA ACC TGG TAC CCA GAG CAG CAG TAC CCA TAG CAG GAG TGT GTC TGT CTC CAT GGT GG-3′ (Metabion, Martinsried, Germany) and cloned into the pcDNA5/FRT vector (Thermo Fisher Scientific Inc., Waltham, MA, USA) in frame with the codons for 6 histidine residues (6 × His-tag) at the 3′-end to facilitate purification of the recombinant protein. Finally, this construct was inserted into the NheI and NaeI site of the expression vector pTT5 (National Research Council of Canada, Quebec, Canada). A self-cleavage-resistant form of mouse neutrophil elastase was made with the help of the oligoduplex DJ3395 5′-Pho-GTG AAC GTA TGC ACT CTG GTG CCA CGT CGA AAG GGT GGC ATC TGC TTC GGG GAC TCT-3′ and DJ3396 5′-Pho-A GTC CCC GAA GCA GAT GCC ACC CTT TCG ACG TGG CAC CAG AGT GCA TAC GTT CAC AC-3′, changing the residues Gln187–Ala188 of mouse neutrophil elastase to Lys187–Gly188. All proteins were expressed in HEK293 EBNA cells (Yves Durocher, National Research Council Canada, Montreal, Canada) that were grown as suspension culture in FreeStyleTM 293 expression medium (Thermo Fisher Scientific Inc.), 1% Pluronic and G418 (25 μg ml −1 ) at 37 °C and 8% CO 2 . Cells were transfected using polyethylenimine–DNA complexes. Elastase variants were purified using PrepEase Histidine-tagged Protein Purification Midi Kit—High Specificity (Affymetrix, Santa Clara, USA) according to the manufacturer’s instructions. Determination of active mouse neutrophil elastase Trypsin was burst titrated in veronal buffer with 4-nitrophenyl 4-guanidinobenzoate (Sigma-Aldrich, St Louis, USA) [28] and then used for the titration of AAT. Different concentrations of standardized AAT (Athens Research & Technology, Athens, GA, USA) were incubated with a constant volume of mouse neutrophil elastase at 37 °C for 1 h. Thereafter, the residual activity was measured. The tc mouse neutrophil elastase was titrated using 1 mM Boc-Ala-Pro-Nva-4-chloro-SBzl (Bachem, Bubendorf, Switzerland) together with 0.5 mM 5′,5′-dithio-bis(2-nitrobenzoic acid), while 0.5 mM MeOSuc-AAPV-pNA substrate was used for the measurement of sc mouse neutrophil elastase activities. All reactions were performed in 150 mM NaCl, 50 mM Tris, 0.01% Triton-X-100, pH7.4. The absorbance was monitored at a wavelength of 405 nm and 22 °C. K m and catalytic rate constant k cat Active mouse neutrophil elastase concentrations for the determination of the Michaelis–Menten constant ( K m ) were either 23 nM sc mouse neutrophil elastase or 231 nM tc mouse neutrophil elastase. Concentrations of the substrates ([S]) MCA-GEAIPMSIPPEVK(Dnp)-rr (EMC microcollections, Tübingen, Germany) were varied between 1 and 80 μM and plotted against reaction rate. Data were fitted to the Michaelis–Menten equation using GraphPad Prism (GraphPad Software Inc., La Jolla, USA). In case all enzymes bind substrates, the catalytic rate constant ( k cat ) is obtained with equation (1). [E] is the total enzyme concentration. The fluorescence was measured at 405 nm after excitation at 320 nm. Inhibitor constants In the presence of a competitive inhibitor (I), the Michaelis–Menten kinetics are given by equation (2). Initial enzyme reaction rates ( v 0 ) were determined as a function of the substrate concentration in the absence and presence of five different inhibitor concentrations ([I]). The inhibition constant K i was determined from these curves using GraphPad (GraphPad Software Inc.). For irreversible inhibition, inhibitor constants were obtained using the conditions described by Duranton and Bieth [29] . To avoid substrate depletion, [S] was five times higher than K m . To keep [I] constant, [I] was at least five times higher than the enzyme concentration. mNE (10 nM) was added to a mix of 60–700 nM of inhibitor and 152 μM substrate MCA-GEAIPTSIPPEVK(Dnp)-rr (EMC microcollections GmbH, Tübingen, Germany). The fluorescence progression curve was recorded immediately (excitation 320 nm, emission 405 nm) thereafter. Using GraphPad Prism, the progression curves were fitted to equation (3) and the observed Michaelis–Menten constant ( k obs ) was obtained. Plotting k obs against the inhibitor concentration and fitting it to equation (4) (GraphPad Prism), the apparent inhibitor constant ( K i(app) ) was determined. The association rate constant ( K ass ) was derived from equation (5). Identification of neutrophil elastase in biological samples Isolated PMNs from the peripheral blood were lysed in RIPA-buffer (30 mM Tris-HCl pH8, 150 mM NaCl, 0.5% deoxycholate, 0.1% SDS, 1% IGEPAL CA-630, 1 mM EDTA) in the presence of 20 nM biotinylated AAPV-chloromethyl ketone inhibitor. Inhibited human neutrophil elastase was captured with 8 μg anti-human neutrophil elastase antibodies (QED Biosciences Inc., San Diego, USA, Cat. No.12303) at 4 °C after overnight incubation. Protein G dynabeads (Life technologies, Invitrogen) were used according to the manufacturer’s instructions to isolate the antibody–antigen complexes. Making use of the biotinylated AAPV-chloromethyl ketone, active human neutrophil elastase was detected with streptavidin-HRP after the precipitate was separated by SDS–PAGE and blotted. Sputum derived human neutrophil elastase (Elastin Products Company, Owensville, MO, USA) was used as a control. Murine PMNs were isolated from the bone marrow of female 129S6/SvEv mice (wild type and PR3/NE-deficient) aged 8–10 weeks and directly boiled in Laemmli sample buffer at 95 °C under reducing conditions. Western blotting after SDS–PAGE was performed with anti-NE antibodies (Abcam; Cambridge, UK, ab68672, dilution 1:1,000) and secondary peroxidase-conjugated anti-rabbit antibodies (Jackson Immunoresearch Laboratories, USA; cat. No. 111-035-006, dilution 1:5,000). Animal experiments Female C57BL/6 mice, 8–10 weeks old, were treated with sc neutrophil elastase or tc neutrophil elastase in 80 μl volume per mouse (4 mg protease per kg body weight) by an oropharyngeal mode. Control mice ( n =3) received 80 μl sterile buffer (300 mM NaCl, 20 mM Na 2 HPO 4 pH7.4). Mice were killed after 2 months for the long-term experiments. The animal study was repeated twice with four mice in each mouse neutrophil elastase group. For the analysis of cell influx and chemokine levels, the mice were killed after 24 h. The animal study was performed twice with four mice in both tc neutrophil elastase and buffer control groups and three and four mice in the sc neutrophil elastase groups. All experiments were conducted under strict governmental and international guidelines and were approved by the local government for the administrative region of Upper Bavaria. Embedding and staining Left lungs were inflated with 6% paraformaldehyde in PBS at 20 cm H 2 O pressure. To obtain systematic uniform random sampling, the lung block embedded in agar, was cut into 2 mm thick slices using a tissue matrix. Afterwards the lung slices were embedded in paraffin and stained with haematoxylin and eosin. Morphometry An Olympus BX51 light microscope equipped with a computer-assisted stereological toolbox (NewCAST of Visiopharm, Hoersholm Denmark) was used to analyse the lung sections. A line grid was superimposed on images of lung section at × 20 objective. Intercepts of lines with alveolar septa and points hitting airspace were counted to calculate mean chord length (MCL) applying the formula: MCL=∑Pair × L(p)/∑Iseptax 0,5; where, ∑Pair=sum points of the grid hitting air spaces, L(p)=line length per point, ∑Isepta=sum of intercepts of alveolar septa with grid lines. Histological scoring The severity of lung inflammation was scored by examining haematoxylin and eosin-stained lung sections using a five-point lung inflammation scoring system. Each lung was scored on each slide at a magnification of 20-fold. Within each field, inflammatory cells were assigned according to predominated criteria—0, no inflammation; 1, <5 inflammatory cells per field; 2, 6–10 inflammatory cells per field; 3, 10–20 inflammatory cells per field; 4, 20–30 inflammatory cells per field; 5, >30 inflammatory cells per field. Preparation of BAL BAL was obtained to analyse the total and differential cell counts for inflammatory cell recruitment of neutrophils and macrophages. The lungs were lavaged by instilling the lungs with 2 × 0.5 ml aliquots of sterile PBS (Gibco, Life Technologies, Darmstadt, Germany). For cytospins, cells were spun down at 400 g for 20 min and resuspended in RPMI-1640 medium containing 10% fetal calf serum (both from Gibco). Total cell counts were determined in a haemocytometer. Differential cell counts were performed using morphological criteria on May–Grünwald–Giemsa-stained cytospin slides (200 cells per sample). BAL fluid was used to evaluate cytokine secretion. Measurement of cytokines and chemokines Monocyte chemotactic protein 1 (MCP1/CCL2) and keratinocyte chemoattractant (KC/CXCL1) levels were determined in BAL fluid using commercially available ELISA kits (R&D Systems Europe, Abingdon, UK) according to the manufacturer’s instructions. In brief, a 96-well microplate was coated with diluted capture antibody (100 μl per well) and incubated overnight at room temperature (RT). Followed by blocking with reagent diluent (1% bovine serum albumin in PBS, pH 7.2–7.4) at RT for 1 h, the sample or standard was added to each well and incubated at RT for 2 h. Next, the plate was incubated with detection antibody diluted in reagent diluent at RT for 2 h. Subsequently, a working dilution of Streptavidin-HRP was added to each well and incubated for 20 min at RT in the dark. Next, the plate was incubated with substrate solution at 1:1 ratio of colour reagent A H 2 O 2 and colour reagent B (tetramethylbenzidine) also for 20 min at RT in the dark. Finally, 50 μl of stop solution (2 N H 2 SO 4 ) was added. The plate was gently tapped to ensure thorough mixing. Optical density was determined immediately, using a microplate reader set to 450 nm. Of note, each incubation step is followed by washing three times with wash buffer (0.05% Tween 20 in PBS, pH 7.2–7.4). Statistics Results are given as mean values±s.e.m. The one-way analysis of variance Bonferroni test was applied in all studies (* P <0.05, ** P <0.01, *** P <0.001). Analyses were conducted by use of GraphPad Prism 6 software (GraphPad Software). How to cite this article: Dau, T. et al . Autoprocessing of neutrophil elastase near its active site reduces the efficiency of natural and synthetic elastase inhibitors. Nat. Commun . 6:6722 doi: 10.1038/ncomms7722 (2015).